RETRACTED ARTICLE: Supported black phosphorus nanosheets as hydrogen-evolving photocatalyst achieving 5.4% energy conversion efficiency at 353 K Solar-driven water splitting using powdered catalysts is considered as the most economical means for hydrogen generation. However, four-electron-driven oxidation half-reaction showing slow kinetics, accompanying with insufficient light absorption and rapid carrier combination in photocatalysts leads to low solar-to-hydrogen energy conversion efficiency. Here, we report amorphous cobalt phosphide (Co-P)-supported black phosphorus nanosheets employed as photocatalysts can simultaneously address these issues. The nanosheets exhibit robust hydrogen evolution from pure water (pH = 6.8) without bias and hole scavengers, achieving an apparent quantum efficiency of 42.55% at 430 nm and energy conversion efficiency of over 5.4% at 353 K. This photocatalytic activity is attributed to extremely efficient utilization of solar energy (~75% of solar energy) by black phosphorus nanosheets and high-carrier separation efficiency by amorphous Co-P. The hybrid material design realizes efficient solar-to-chemical energy conversion in suspension, demonstrating the potential of black phosphorus-based materials as catalysts for solar hydrogen production. The global energy crisis is increasingly spotlighting, causing many serious issues, such as climate change, food safety, human health, etc. [1] , [2] . Development and use of clean energy have been extremely urgent to circumvent these issues. It is well known that H 2 is one of the cleanest and most promising energy resources because of its high-energy capacity of 143 MJ kg −1 and emission-free feature [3] , [4] , [5] . However, most of hydrogen fuel is obtained via the steam-reformed methane process today, where a substantial amount of CO 2 is generated because of the consumption of fossil fuels [6] . As an alternative, photocatalytic water splitting using solar energy and powdered catalysts shows to be promising for green production of H 2 , independent of fossil reserves [7] , [8] . Following the pioneering study of water splitting over a TiO 2 electrode reported in 1972, lots of efforts have been devoted to solar-driven water splitting during the past decades [9] , [10] , [11] . However, it is still challenging to realize practicable solar-to-hydrogen conversion efficiency (STH) in suspension systems [12] . Generally, light harvesting capability and carrier separation efficiency are especially crucial, determining the activity of photocatalysts [13] , [14] . The last decades have witnessed the success of extending light-absorption capability of photocatalysts from visible to near-infrared by bandgap engineering and plasmon coupling [15] , [16] . Unfortunately, most of these catalysts were operated with the assistance of sacrificial reagents, associated with the rapid recombination of photogenerated carriers. Therefore, the kinds of photocatalysts used for steady visible-light-driven-overall water splitting are still very limited to date [17] . In principle, overall water splitting consists of water reduction and oxidation half-reactions, where water oxidation half-reaction provides a large-scale source of electrons and protons for water reduction, but showing slow kinetics owing to complicated four-electron reaction process and huge activation energy barrier for the formation of O−O bond, therefore, obstructing the large-scale hydrogen production [18] . As one of phosphorus allotropes, black phosphorus (BP) is a fascinating two-dimensional material, consisting of corrugated planes of phosphorus atoms with strong intralayer bonding and weak interlayer interactions and showing thickness-tunable bandgap from 0.46 to 1.51 eV, as well as highly free-carrier mobility [19] . These unique properties render few-layer BP nanosheets promising as photocatalyst for hydrogen production. For example, Zhu et al. [20] demonstrated the hydrogen evolution from water by BP nanosheets with excellent stability. Very recently, electron transfer was studied in g-C 3 N 4 -supported BP nanosheets, showing that BP nanosheets are suitable candidate as photocatalyst for solar water splitting [21] . Lack of wet-chemical approach toward the preparation of few-layer BP nanosheets, however, is restricting the further development of BP-based materials as photocatalysts for water splitting [22] , [23] . Herein, we demonstrate that one-pot solvothermal process is feasible for the direct preparation of few-layer BP nanosheets. After loading amorphous cobalt phosphide (Co-P) nanoparticles as cocatalyst, the supported BP nanosheets achieve scalable hydrogen evolution from pure water with an apparent quantum efficiency (AQE) of 42.55% at 430 nm and STH efficiency of over 5.4% at 353 K. Moreover, we find that ·O 2 − , ·OH, and H 2 O 2 are formed as products of water oxidation via two-electron process instead of more difficult four-electron process for O 2 formation in the system, combining efficient separation of electron–hole pairs by amorphous Co-P nanoparticles, responsible for the robust hydrogen production from pure water. Preparation and characterization of BP-based samples At present, the majority of few-layer BP nanosheets are prepared via the mechanical or solution-based exfoliation of bulk BP, which is time consuming and costly because it is not easy to synthesize bulk BP and BP degrades rapidly when exfoliated to nanoscale dimensions [19] , [20] , [21] , [22] , [23] . Here, a direct solvothermal reaction of white P in ethylenediamine, without any additives, is run for the preparation of few-layer BP nanosheets. To improve photocatalytic activity, amorphous Co-P nanoparticles are supported on the few-layer BP nanosheets via the same procedure but using Co(NO 3 ) 2 ·6H 2 O as raw material. The mechanism for the formation of amorphous Co-P nanoparticles on BP nanosheets is proposed as follow (Fig. 1a ). Layered red phosphorus is formed initially via the conversion of white phosphorus at room temperature with the assistance of ethylenediamine, which is revealed by Raman and transmission electron microscopy (TEM) characterizations (Supplementary Fig. 1 ). The interaction between layered red phosphorus and ethylenediamine will induce ethylenediamine molecules access to the interlamination of layered red phosphorus. As a result, the interlamellar spacing increases and the van der Waals’ force of interlamination decreases [24] . With the help of heating as driving force, the layered red phosphorus nanosheets are exfoliated to be few-layer red phosphorus nanosheets. Meanwhile, the further phase transformation from red phosphorus to BP occurs in the exfoliation process. The similar process can be also observed in the conversion from layered α-Co(OH) 2 nanocones to single-layer β-Co(OH) 2 nanosheets [25] . In this whole synthetic process, ethylenediamine plays a critical role. Once few-layer BP nanosheets are formed, free Co 2+ ions will react with them to form amorphous Co-P nanoparticles on the surface of the BP nanosheets [26] . We need to emphasize that the whole synthetic process presented here is much simpler than traditional protocol for the preparation of few-layer BP nanosheets. No special setup and chemicals are used, thus, reducing production costs of BP-based materials greatly. Fig. 1 Spectroscopic characterizations of the as-prepared BP-based samples. a The formation process of the Co-P/BP nanosheets: (1) phase transition processes, (2) supporting process via the reaction between the formed BP nanosheets and Co(NO 3 ) 2 . The reaction was run in ethylenediamine, followed by heating at 140 °C for 12 h, respectively. b XRD patterns of the BP (red line) and Co-P/BP (navy line) samples. c Raman spectra of the pristine BP and Co-P/BP samples. The excitation wavelength is 633 nm. d , e XPS fine spectra of P 2 p and Co 2 p states in the samples. The C 1 s (284.8 eV) is the charged correction benchmark Full size image As shown in Fig. 1b , the product prepared via solvothermal process shows the typical X-ray diffraction (XRD) pattern of the orthorhombic of BP ((Space group: Cmca (64)) and no other phases are detected [27] , suggesting that pure BP is obtained. The weak and broaden XRD peaks reveal the low crystallinity and small size, which are beneficial for the improvement of photocatalytic activity because much more defects are easily formed in the samples prepared via wet-chemical route [28] . After supporting, we cannot observe the XRD signals from Co-related species, but energy dispersive X-ray spectroscopy (EDX) (Supplementary Fig. 2 ) clearly confirms the existence of Co in addition to P in the sample. Inductively coupled plasma-atomic emission spectral (ICP-AES) analysis further reveals that the mass ratio of P to Co is around 8 (Supplementary Fig. 3 ). In addition, we can also find that the diffraction peak of (020) shifts to the small-angle side after supporting, which should be attributed to the interaction between BP nanosheets and the supporting Co-based material [29] . Raman spectra of the samples exhibit the similar spectral profiles, consisting of four Raman peaks between 300 and 500 cm −1 (Fig. 1c ). Typically, three of them are characteristic Raman peaks of BP: A 1 g (365 cm −1 ), B 2g (442 cm −1 ), and A 2 g (470 cm −1 ) [30] , which further suggest that BP nanosheets can be prepared via the protocol developed here. The peak at 388 cm −1 should be assigned to the characteristic peak of P–O bond because of oxidation of P (Supplementary Fig. 4). The surface chemical states of the samples are characterized by X-ray photoelectron spectroscopy (XPS). As shown in Fig. 1d , both 2 p 3/2 (129.9 eV) and 2 p 1/2 (130.8 eV) states can be observed in BP and supported BP, suggesting the same chemical state of P atoms in these two samples [17] . However, another P signal at binding energy of 129.5 eV is detected in the supported sample, assignable to P atom in phosphide cobalt [29] . Moreover, two well-formed peaks at 779.9 and 795.0 eV are found in Co 2 p spectrum for the supported sample (Fig. 1e ), which are consistent with Co XPS signals in Co-P [31] , [32] . Therefore, we can conclude that few-layer BP nanosheets are supported by amorphous Co-P nanoparticles. In addition, a broad XPS band deconvoluted into three peaks at 131.8 and 133.2 eV can be observed in P 2 p spectra for these samples, attributed to P–O–P and P=O [20] , respectively, which is further confirmed by O 1 s XPS spectrum (Supplementary Fig. 5 ). Typically, there are two intense peaks at 530.8 and 532.4 eV in O 1 s XPS spectrum, which is assigned to P=O and P–O–P bonds, respectively [20] . Although the inevitable oxidation occurred in our samples, the oxidation was confirmed to be beneficial for the improvement of the stability of BP [33] . The morphology and structure of the as-prepared BP-based samples are studied by TEM. Fig. 2a shows that the as-prepared Co-P/BP consists of a nanosheet structure, where amorphous Co-P nanoparticles of around 5 nm in diameter are supported on the BP nanosheets. The high-resolution TEM image (HRTEM) clearly shows the crystal lattice of the nanosheets, corresponding to 0.507 nm d -spacing of the (020) plane of orthorhombic BP (Fig. 2b ). However, crystal lattices cannot be observed in the Co-P nanoparticles, suggesting an amorphous structure, which is in line with the XRD results. The typical nanosheet structure also can be observed in the TEM image of the as-prepared BP sample (Supplementary Fig. 6 ). Furthermore, element mapping results (Fig. 2c ) indicate that the amount of P is more than that of Co, which is consistent with the result from ICP-AES as well. All results confirm that amorphous Co-P nanoparticles are supported on the BP nanosheets. In addition, atomic force microscopy was implemented to study the thickness of the as-prepared supported BP nanosheets. As shown in Fig. 2d, e , we can see that the as-prepared sample has an obvious nanosheet structure with a thickness about 1.4 nm (about 2−3 layers) [34] . Fig. 2 Morphology and structure of the Co-P/BP nanosheets. a , b TEM and HRTEM images of the Co-P/BP nanosheets. The red circles marked are amorphous Co-P nanoparticles and the nanosheet structure is BP. c EDX element mapping. The high-angle annular dark fields (HAADF) scanning transmission electron microscope (STEM) of the region of interest, as well as Co and P distribution, are shown. d , e AFM image and the corresponding height profiles of the Co-P/BP nanosheets. The scale bars are 50, 5, 40, and 20 nm in Fig. 2a, b, c, and d , respectively. In all panels, the mass ratio of P to Co is about 8 Full size image Bandgap states of the Co-P/BP nanosheets Effective harvesting of sunlight is necessary for driving photocatalytic reactions. To reveal the harvesting capability of sunlight, therefore, the absorption spectra of the BP-related samplers are measured by diffuse reflectance ultraviolet–visible–near-infrared (UV–vis–NIR) spectroscopy. As shown in Fig. 3a , the absorption edge of the as-prepared BP nanosheets is around 1013 nm, corresponding to a bandgap energy of 1.16 eV [34] . After supporting amorphous Co-P nanoparticles, a slight increase of absorption in NIR can be observed, which is probably caused by low levels of crystallinity and defects in the prepared amorphous Co-P nanoparticles and the electronic coupling between BP nanosheets and amorphous Co-P nanoparticles [35] , [36] . A bandgap energy was deduced to be 1.14 eV for the Co-P/BP nanosheets by the plots (Fig. 3b ). Based on their light-absorption features, the as-prepared BP and Co-P/BP nanosheets, exhibiting sufficient capability of harvesting solar light (~75% of solar energy), should be active photocatalysts under UV–vis–NIR irradiation. Fig. 3 Bandgap states of the as-prepared BP-based samples. a UV–vis–NIR absorption spectra of the BP (red curve) and Co-P/BP (navy curve) nanosheets. The inset is digital photographs of the as-prepared samples. b ( ahν ) 2 vs. hν curve for BP (red curve) and Co-P/BP (navy curve) nanosheets. The dashed lines are the tangents to the curves. The intersection value is the bandgap. c Mott–Schottky plots for the BP and Co-P/BP nanosheets from impedance measurements. The flat-band potentials were obtained from the intercepts of the extrapolated lines. d Band positions of the BP and Co-P/BP nanosheets from the bandgaps and flat-band potentials obtained from Fig. 3c Full size image To further determine the relative band structure of the BP-based nanosheets, XPS valence band (VB) spectra and flat-band potential were measured. According to the XPS valence spectra (Supplementary Fig. 7 ), the VB energy levels of BP and Co-P/BP nanosheets are estimated to be ~0.51 and ~0.48 eV below the Fermi level. The Mott–Schottky plots exhibit a negative slope, suggesting the nature of p-type semiconductor of BP nanosheets (Fig. 3c ) [37] . Further, the flat-band potentials ( E FB , approximate to the Fermi level) of BP and Co-P/BP nanosheets are estimated to be −0.11 and −0.10 V (vs. reverse hydrogen electrode (RHE)). Based on the known bandgap of the BP (1.16 eV) and Co-P/BP nanosheets (1.14 eV), the conduction band (CB) and VB energy levels of BP nanosheets are calculated to be −0.76 and 0.40 V vs. RHE, while the CB and VB energy levels of Co-P/BP nanosheets are calculated to be −0.76 and 0.38 V vs. RHE. Therefore, the as-prepared BP and Co-P/BP nanosheets are only suitable for extracting hydrogen from water as their conduction band positions are on the top of the reduction potential of H 2 O/H 2 and VB positions are at the bottom of the oxidation potential of O 2 /H 2 O (Fig. 3d ). Photocatalytic hydrogen evolution from pure water The experiments of photocatalytic hydrogen evolution from pure water (pH = 6.8, without sacrificial reagents) were carried out in an air-tight flask under Xe lamp irradiation ( λ ≥ 420 nm) at ambient pressure. Typical H 2 and O 2 signals are detected simultaneously by gas chromatography (GC) (Supplementary Fig. 8 ), but with the ratio not as expected 2:1. We find that the production rate of H 2 increases as the intensity of incident light increases (Supplementary Fig. 9 ), suggesting that H 2 production over the Co-P/BP nanosheets is a photocatalytic process rather than a self-corrosion reaction. Hydrogen bubbles are also observed obviously over the Co-P/BP nanosheets immersed in pure water under Xe lamp irradiation, as presented in Supplementary Movie 1 . In order to further confirm the detected H 2 and O 2 from water, H 2 O was replaced by 4 H 2 O and H 2 18 O as solvents in photocatalytic reaction system, respectively. GC–mass spectrometry results reveal that 4 H 2 is mainly hydrogen specie when 4 H 2 O is used, while a small number of 18 O 2 specie is detected when H 2 18 O was used (Supplementary Fig. 10 ), indicating that photocatalytic water splitting reaction indeed occurs in our system. The dependence of H 2 evolution rate on the concentration of the catalyst was determined first in the system, showing that the optimal amount of the catalyst is 40 mg for achieving the maximal H 2 evolution rate (Supplementary Fig. 11 ). Figure 4a shows the time courses for H 2 evolution over the BP and Co-P/BP catalysts (In Co-P/BP sample, the mass ratio of P to Co is 3) irradiated by Xe lamp ( λ ≥ 420 nm, 100 mW cm −2 ) for 2 h. The H 2 -evolving rate of the as-prepared BP nanosheets is determined to be 1.2 μmol h −1 . After supporting amorphous Co-P nanoparticles, the supported BP nanosheets exhibit a H 2 -evolving rate of 15 μmol h −1 , which is around 12-fold improvement compared to the unsupported BP nanosheets. The improvement of activity should be associated with low recombination of electron–hole pairs induced by amorphous Co-P nanoparticles as cocatalyst, which is further confirmed by the electrochemical results (Supplementary Figs. 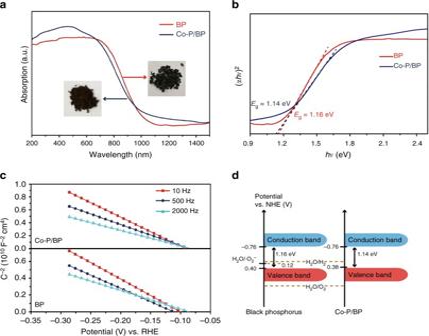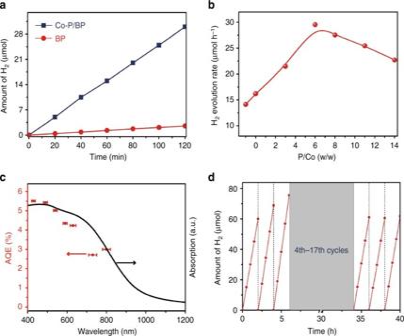Fig. 4 Photocatalytic H2evolution over the BP-based catalysts.aTypical time courses of H2evolution over the BP and Co-P/BP nanosheets under Xe lamp illumination (PLS-SXE300C,λ≥ 420 nm). The mass ratio of Co to P is 1/3.bEffect of the mass ratio of Co to P on the photocatalytic activity in the Co-P/BP nanosheets.cWavelength-dependent AQE (red squares) of H2evolution over the optimal Co-P/BP catalyst irradiated by a 300-W Xe lamp using a bandpass filter ofλ± 10 nm for 430, 490, 540, and 590 nm;λ± 15 nm for 630 nm;λ± 30 nm for 730 and 800 nm. The errors bars represent wavelength error of filters.dStability of photocatalytic H2evolution over the Co-P/BP catalyst in pure water. For all the photocatalytic water-splitting experiments, 40 mg of the catalyst was dispersed in 150 mL pure water (pH = 6.8) followed irradiation by 300-W Xe lamp with output power of 100 mW cm−2 Fig. 3 Bandgap states of the as-prepared BP-based samples.aUV–vis–NIR absorption spectra of the BP (red curve) and Co-P/BP (navy curve) nanosheets. The inset is digital photographs of the as-prepared samples.b(ahν)2vs.hνcurve for BP (red curve) and Co-P/BP (navy curve) nanosheets. The dashed lines are the tangents to the curves. The intersection value is the bandgap.cMott–Schottky plots for the BP and Co-P/BP nanosheets from impedance measurements. The flat-band potentials were obtained from the intercepts of the extrapolated lines.dBand positions of the BP and Co-P/BP nanosheets from the bandgaps and flat-band potentials obtained from Fig.3c 12 − 17 ). Furthermore, the amount of amorphous Co-P nanoparticles is found to have a substantial effect on activity of the catalyst (Fig. 4b ). Clearly, the highest H 2 -evolving activity is obtained at the mass ratio of P to Co of 8 (29.4 μmol h −1 ). Further increasing the ratio of P to Co leads to the decrease of activity because overloading of amorphous Co-P nanoparticles on the surface of BP nanosheets would lead to the decrease of light absorption [38] . For a more objective evaluation of photocatalytic activity for hydrogen production by the Co-P/BP nanosheets, the AQE of the Co-P/BP nanosheets with a mass ratio of P to Co of 8 were measured under monochromatic light radiation ( λ = 430, 490, 540, 590, 630, 730, and 800 nm). The results show an excellent correlation between the absorption spectrum and AQE in the Co-P/BP nanosheets, indicating H 2 evolution is induced by excitation of BP nanosheets (Fig. 4c ). The highest AQE of 5.50% is obtained at λ = 430 nm at room temperature. With the increase of wavelength of incident light, AQE decreases, however, the increase of AQE can be observed at 800 nm, which can be attributed to the thermal effect induced by near-infrared light, leading to increase the rate of hydrogen evolution in kinetics. Fig. 4 Photocatalytic H 2 evolution over the BP-based catalysts. a Typical time courses of H 2 evolution over the BP and Co-P/BP nanosheets under Xe lamp illumination (PLS-SXE300C, λ ≥ 420 nm). The mass ratio of Co to P is 1/3. b Effect of the mass ratio of Co to P on the photocatalytic activity in the Co-P/BP nanosheets. c Wavelength-dependent AQE (red squares) of H 2 evolution over the optimal Co-P/BP catalyst irradiated by a 300-W Xe lamp using a bandpass filter of λ ± 10 nm for 430, 490, 540, and 590 nm; λ ± 15 nm for 630 nm; λ ± 30 nm for 730 and 800 nm. The errors bars represent wavelength error of filters. d Stability of photocatalytic H 2 evolution over the Co-P/BP catalyst in pure water. For all the photocatalytic water-splitting experiments, 40 mg of the catalyst was dispersed in 150 mL pure water (pH = 6.8) followed irradiation by 300-W Xe lamp with output power of 100 mW cm −2 Full size image In addition to extraordinarily photocatalytic activity, Co-P/BP nanosheets also exhibit excellent stability as a photocatalyst. No obvious decrease in the photocatalytic activity for hydrogen production is observed in the cycling tests (Fig. 4d ). The photocatalytic activity is maintained well within at least 40 h of illumination. To further verify the stability of the catalyst, XRD, TEM, and XPS were performed after the photocatalytic reaction. There were no obvious changes in the crystal structure, morphology, and surface chemical states of the catalyst (Supplementary Figs. 18 – 20 ), indicating that the Co-P/BP catalyst possesses good stability. Besides good photocatalytic activity in pure water (pH = 6.8), the Co-P/BP catalyst shows good activity in the broad pH range from 2 to 13 (Supplementary Fig. 21 ). STH efficiency is one of most vital indexes for evaluating the performance of catalysts. However, STH value is rarely reported because most of catalysts exhibit negligible hydrogen evolution activity in pure water. Over the recent decade, scientists have put forward new strategies to improve photocatalytic water-splitting performance of catalysts, such as plasmon coupling, bandgap engineering, etc. 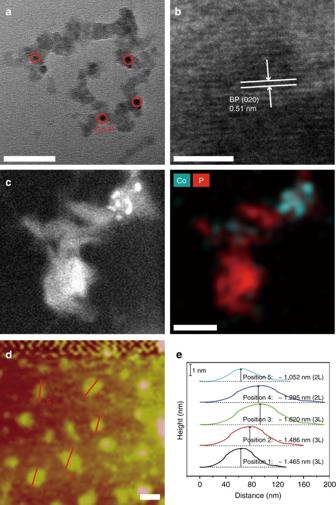[39] , [40] , [41] . These methods do work well but only with the assistance of sacrificial reagents. Fig. 2 Morphology and structure of the Co-P/BP nanosheets.a,bTEM and HRTEM images of the Co-P/BP nanosheets. The red circles marked are amorphous Co-P nanoparticles and the nanosheet structure is BP.cEDX element mapping. The high-angle annular dark fields (HAADF) scanning transmission electron microscope (STEM) of the region of interest, as well as Co and P distribution, are shown.d,eAFM image and the corresponding height profiles of the Co-P/BP nanosheets. The scale bars are 50, 5, 40, and 20 nm in Fig.2a, b, c, and d, respectively. In all panels, the mass ratio of P to Co is about 8 Photocatalytic water splitting using particulate semiconductors still suffers from low-energy conversion efficiency [42] . In this study, we obtained STH efficiency in the Co-P/BP system via loading 40 mg of the Co-P/BP catalyst in 150 mL pure water under AM1.5 G simulated sunlight illumination (100 mW cm −2 ). About 160 μmol of H 2 was generated after 2 h of irradiation. The total incident power over the irradiation area of 8 cm 2 was 0.8 W, so the STH efficiency of the Co-P/BP catalyst with the optimal ratio of Co to P of 8 was determined to be about 0.66% at room temperature—a high-STH value compared to previously reported catalysts operated in pure water [43] , [44] , [45] , [46] , [47] . As mentioned above, temperature has a great effect on the photocatalytic activity of hydrogen evolution over the Co-P/BP nanosheets. To further confirm this, we studied the temperature-dependent photocatalytic activity over the Co-P/BP nanosheets in pure water. As shown in Fig. 5a , the hydrogen-evolving rate is improved monotonically from 29.4 to 131.6 µmol h −1 as the temperature increases from 298 to 353 K at an ambient pressure. The activation energy for the hydrogen evolution over the Co-P/BP nanosheets was deduced to be 32.8 kJ mol −1 (inset in Fig. 5a ), which is smaller than that of electrochemical H 2 evolution from acidic or basic solutions [48] . The activation energy is a key indicator, reflecting whether photocatalytic H 2 evolution occurs easily [48] . Usually, the lower activation energy is, the easier photocatalytic H 2 evolution occurs. Therefore, a low-activation energy in our system indicates that the hydrogen evolution is easier. The AQE for hydrogen evolution reach 42.55% at 430 nm, accompanied by a STH value of 5.4% at 353 K and 101 kPa (Fig. 5b ). Very recently, an exciting AQE of 33% at 419 nm and STH of 1.1% were achieved in Z-scheme catalyst based on SrTiO 3 :La, Rh/Au/BiVO 4 :Mo at 331 K and 10 kPa 2 . By comparison, the amorphous Co-P nanoparticles supported BP nanosheets, definitely, records by far the highest AQE and STH amongst the photocatalytic hydrogen-evolving systems based on powdered semiconductors without any external assistance. The Department of Energy of the United State reported that the STH efficiency target for photocatalytic water splitting is 5% in 2020 for realistic application, allowing the cost of $4.6 kg −1 for hydrogen generation, which is much cheaper than that from the photoelectrochemical process [12] . Therefore, BP-based materials show to be promising as photocatalysts for solar-hydrogen production. Additionally, the photocatalytic activity of the Co-P/BP nanosheets was also explored to split seawater, because seawater is the most abundant and geographically balanced natural water resource available on earth. The hydrogen evolution rate is a 6.8 μmol h −1 in seawater (Supplementary Fig. 22 ). Moreover, after 20 cycles, the photocatalytic activity was maintained well. These results confirm the Co-P/BP nanosheets have good activity and photostability in seawater. Compared to the activity in pure water, however, the activity decreases may because of the large number of ions in seawater. Fig. 5 Temperature-dependent photocatalytic activity over the Co-P/BP nanosheets. a The effect of temperature on hydrogen evolution rate over the Co-P/BP nanosheets at ambient pressure. The inset is Arrhenius plot for determination of the activation energy for hydrogen evolution using Co-P/BP nanosheets as catalyst from pure water (pH = 6.8). The activation energy was deduced to be 32.8 kJ mol −1 . b The STH (blue square) and AQE at 430 nm (red sphere) as a function of temperature over the Co-P/BP nanosheets. The STH was measured under the irradiation of AM 1.5 G simulated solar light (100 mW cm −2 ). In all panels, the mass ratio of P to Co is about 8 Full size image Photocatalytic hydrogen evolution mechanism To confirm that the excellent photocatalytic activity is associated with efficient electron transfer from BP nanosheets to amorphous Co-P nanoparticles besides sufficient capability of harvesting light of the BP nanosheets. The transient absorption spectra (TAS) of the BP and Co-P/BP nanosheets were measured. As shown in Fig. 6 , we can see that the transient absorption spectra of the surface-trapped holes and electrons in both BP and Co-P/BP nanosheets show a broad NIR absorption band (800–1500 nm) [49] . Typically, as shown in Fig. 6a , we can find that the concentration of photogenerated carriers decays with the time extension, which is attributed to the recombination of the photogenerated electrons and holes in BP nanosheets. A similar positive TAS feature is also observed in the Co-P/BP nanosheets (Fig. 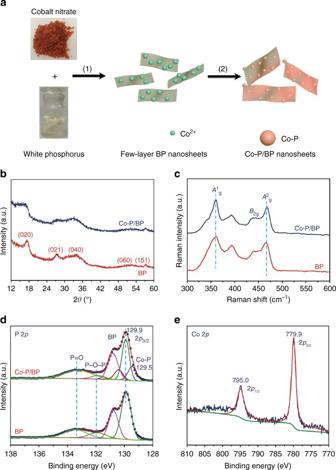6b ), indicating the essentially almost same transient species and trapped electrons [50] . However, the decrease of absorption signal intensity in Co-P/BP nanosheets is much faster than that in unsupported BP nanosheets, which should be attributed to the fast transfer electron from BP to amorphous Co-P nanoparticles. In order to confirm this speculation, the time profiles of the TAS at 1020 nm in BP and Co-P/BP nanosheets are measured (Fig. Fig. 1 Spectroscopic characterizations of the as-prepared BP-based samples.aThe formation process of the Co-P/BP nanosheets: (1) phase transition processes, (2) supporting process via the reaction between the formed BP nanosheets and Co(NO3)2. The reaction was run in ethylenediamine, followed by heating at 140 °C for 12 h, respectively.bXRD patterns of the BP (red line) and Co-P/BP (navy line) samples.cRaman spectra of the pristine BP and Co-P/BP samples. The excitation wavelength is 633 nm.d,eXPS fine spectra of P 2pand Co 2pstates in the samples. The C 1s(284.8 eV) is the charged correction benchmark 6c ), and their average lifetimes are listed in Supplementary Table 1 . We can see that the average lifetime of the BP nanosheets is about 37.7 ps, which is much longer than that of the Co-P/BP nanosheets (10.2 ps), suggesting that an efficient photogenerated electron transfer from photoabsorber (BP nanosheets) to cocatalyst (Co-P nanoparticles) [51] . Moreover, such remarkable decrease of lifetime after the modification of Co-P nanoparticles further indicates that Co-P nanoparticles is a promising cocatalyst for charge transfer, enhancing photocatalytic hydrogen-evolution activity under light irradiation finally. Fig. 6 Dynamics for the interfacial electron migration in the Co-P/BP nanosheets. a TAS spectra of the BP nanosheets. b TAS spectra of the Co-P/BP nanosheets. c Time profiles of the normalized transient absorption at 1020 nm. The data in Fig. 6c were fitting by biexponential function. All the spectra are obtained by the excitation of a 500 nm pulsed laser Full size image In view of the analysis of band structure of the Co-P/BP nanosheets, we have concluded that the Co-P/BP nanosheets can be only used for reducing water into hydrogen. However, our photocatalytic reactions were run in pure water without sacrificial reagents. Therefore, there must be some other species formed from photogenerated holes during the photocatalytic reaction, such as ·O 2 − radicals, ·OH radicals, or H 2 O 2 . To verify our hypothesis, we employed hydroxylamine hydrochloride and safranine T (SFT) as fluorescent indicators to detect the radicals in the system. It is well known that hydroxylamine hydrochloride can be oxidized by ·O 2 − radicals to form nitrite, which reacts with SFT (Supplementary Fig. 23 ). As a result, the fluorescent intensity of SFT would decrease [52] . As shown in Fig. 7a , a fluorescent signal associated with SFT can be detected, followed by a monotonic decrease of intensity with the increase of the irradiation time, indicating the existence of ·O 2 − radicals. Fig. 7 Determination of oxydates of water by photogenerated holes in the system. a Time-dependent fluorescence emission spectra of the SFT reacted with NO 2 − formed from the reaction between hydroxylamine hydrochloride and ·O 2 − in the Co-P/BP suspension system under Xe lamp irradiation ( λ ≥ 420 nm). b Photodegradation activity of RhB under different conditions. Red line: pristine RhB solution; navy line: Co-P/BP and RhB solution; and light blue line: 1 mM benzoquinone and Co-P/BP and RhB solution. The light source is a 300-W Xe lamp ( λ ≥ 420 nm) and irradiation power is 100 mW cm −2 Full size image Another reagent, 1,4-benzoquinone (BQ, a quencher of superoxide radicals), was also introduced in the suspension solution containing the Co-P/BP nanosheets and rhodamine B (RhB) for further confirming the formation of ·O 2 − radicals under illumination. As shown in Fig. 7b , the degradation rate decreased significantly after the introduction of BQ, indicating the generated ·O 2 − radicals were captured by BQ. Thus, oxidation of RhB is suppressed greatly. In addition, the degradation rate of the Co-P/BP/BQ is faster than that of pristine RhB under illumination, which is attributed to generation of holes. These results demonstrate that the photogenerated holes in the VB of the Co-P/BP are powerful enough to oxidize surface-adsorbed hydroxyl groups and water to form ·O 2 − radicals. Interestingly, the color of the solution containing catalyst and pure water changes from colorless to blue when o-tolidine is added after the illumination (Supplementary Fig. 24 ), suggesting that H 2 O 2 is formed in the system as well [53] . Besides H 2 O 2 and ·O 2 − radicals, ·OH radicals were also detected in photocatalytic systems by electron paramagnetic resonance (EPR) measurements (Supplementary Fig. 25 ). The formation of H 2 O 2 and ·OH radicals can be associated with a series of complicated chemical reactions with the assistance of ·O 2 − radicals. Compared to oxygen production via four-electron process, these species are formed easily via two-electron process, beneficial to produce a large-scale source of electrons and protons for water reduction. Therefore, the Co-P/BP nanosheets exhibit robust hydrogen-evolving activity from pure water. Based on above experimental results and analysis, we provide a possible photocatalytic mechanism in our catalyst system described as follow. The photogenerated holes directly oxidize H 2 O to form ·O 2 − radical (Eq. 1 ), accompanying with protons formation, which has been confirmed by the ·O 2 − radical detection experiments. Meanwhile, the formed H + ions are reduced to hydrogen by electrons (Eq. 2 ). As a result, excess H + ions would be formed in the photocatalytic system (Eq. 3 ), which is well consistent with the pH value of the solution after irradiation (pH = 4.8). In addition, the ·O 2 − radical is easily converted into H 2 O 2 and ·HO radical via a series of complicated chemical reactions (Eqs. 4 – 6 ) [54] . Oxygen is generated in the system via the process described in Eq. 5 . 4H_2O + 6h^ + → 8H^ + + 2 ·O_2^ -
 (1) 
    6H^ + + 6e^ - →3H_2
 (2) 
    4H_2O + hν→ 3H_2 + 2 ·O_2^ - + 2H^ +
 (3) 
    ·O_2^ - + H^ + →·HO_2
 (4) 
    ·HO_2 + ·HO_2→H_2O_2 + O_2
 (5) 
    H_2O_2 + hν→2·OH
 (6) In conclusion, we have successfully demonstrated a promising H 2 -evolving photocatalyst based on amorphous Co-P nanoparticles supported BP nanosheets prepared via a facile, low-cost, and scalable solvothermal route. The catalyst exhibits high capabilities of harvesting vis–NIR light and separating electron–hole pairs, achieving a state-of-the-art AQE of 42.55% at 430 nm and STH of over 5.4% for hydrogen evolution from pure water in absence of sacrificial reagents. Instead of O 2 , ·O 2 − , ·OH, and H 2 O 2 were found to be products of the photogenerated holes in the studied photocatalytic systems. This artificial photosynthesis material has significant advantages over traditional water-splitting processes including no explosion risk from hydrogen and oxygen, noble-metal-free, and easy separation of photocatalytic products. The results presented here confirm the potential of BP-based materials as next-generation solar fuel photocatalysts for solar hydrogen production. Preparation of Co-P/BP nanosheets Co-P/BP nanosheets were synthesized by a directly solvothermal process employing white phosphorus and Co(NO 3 ) 2 ·6H 2 O as raw materials and ethylenediamine as solvent. In a typical synthesis process, an amount of white phosphorus and Co(NO 3 ) 2 ·6H 2 O were dissolved in ethylenediamine under vigorously stirring. Then, the solution was transferred to a 50 mL Teflon liner, followed by heating at 140 °C for 12 h. After cooling to room temperature naturally, the product was collected and washed with benzene, ethanol, and distilled water in sequence, followed by drying in vacuum at 60 °C overnight. The preparation protocol of the BP nanosheets is similar with that of the Co-P/BP nanosheets without the use of Co(NO 3 ) 2 ·6H 2 O. Materials characterizations The XRD patterns were collected using a Rigaku B/Max-RB diffractometer with Cu Kα radiation at 40 kV and 40 mA. 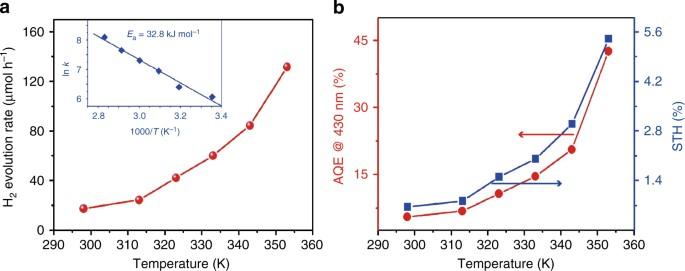Fig. 5 Temperature-dependent photocatalytic activity over the Co-P/BP nanosheets.aThe effect of temperature on hydrogen evolution rate over the Co-P/BP nanosheets at ambient pressure. The inset is Arrhenius plot for determination of the activation energy for hydrogen evolution using Co-P/BP nanosheets as catalyst from pure water (pH = 6.8). The activation energy was deduced to be 32.8 kJ mol−1.bThe STH (blue square) and AQE at 430 nm (red sphere) as a function of temperature over the Co-P/BP nanosheets. The STH was measured under the irradiation of AM 1.5 G simulated solar light (100 mW cm−2). In all panels, the mass ratio of P to Co is about 8 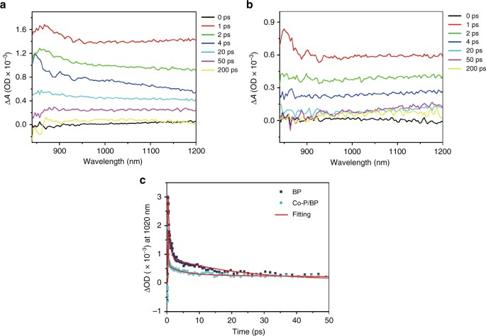Fig. 6 Dynamics for the interfacial electron migration in the Co-P/BP nanosheets.aTAS spectra of the BP nanosheets.bTAS spectra of the Co-P/BP nanosheets.cTime profiles of the normalized transient absorption at 1020 nm. The data in Fig.6cwere fitting by biexponential function. All the spectra are obtained by the excitation of a 500 nm pulsed laser 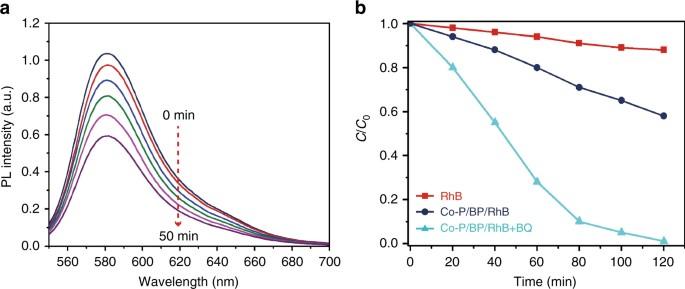Fig. 7 Determination of oxydates of water by photogenerated holes in the system.aTime-dependent fluorescence emission spectra of the SFT reacted with NO2−formed from the reaction between hydroxylamine hydrochloride and ·O2−in the Co-P/BP suspension system under Xe lamp irradiation (λ≥ 420 nm).bPhotodegradation activity of RhB under different conditions. Red line: pristine RhB solution; navy line: Co-P/BP and RhB solution; and light blue line: 1 mM benzoquinone and Co-P/BP and RhB solution. The light source is a 300-W Xe lamp (λ≥ 420 nm) and irradiation power is 100 mW cm−2 TEM and HRTEM images were obtained on a Tecnai-G2-F30 field emission transmission electron microscope with an accelerating voltage of 300 kV. High-angle annular dark fields-scanning transmission electron microscope and EDX maps were recorded on an FEI Titan. XPS analysis was performed on a KRATOS Axis ultra-DLD X-ray photoelectron spectrometer with a monochromatized Mg Kα X-ray source ( hν = 1283.3 eV). AFM was measured using a Veeco DI Nanoscope Multi Mode V system. UV–vis–NIR diffuse reflectance spectra were recorded with a Shimadzu UV-3600 UV–vis–IR spectrophotometer, in which BaSO4 was used as a reflectance standard. Micro-Raman spectra were measured using a LabRam HR800 Jobin-Yvon spectrometer with an excitation wavelength of 633 nm. Ultrafast transient absorption measurements were carried out using a Helios spectrometer (Ultrafast Systems). An amplified Ti:Sapphire pulse (1500 nm, 80 fs, 1.67 kHz repetition rate utilizing a Spectra-Physics Spitfire Pro) was split into two beams. Photocatalytic H 2 evolution from pure water Photocatalytic experiments were carried out in a sealed Pyrex flask (150 mL) with a flat window and a silicone rubber septum for sampling. Typically, 40 mg of the catalyst was added into 150 mL of pure water (pH = 6.8). Subsequently, the suspension was ultrasonicated for 5 min until the powder was dispersed completely. Prior to visible-light irradiation, the flask was degassed by bubbling Ar gas for 30 min. Three hundred watts Xe lamp was used as light source (the output power is fixed as 100 mW cm −2 ), which is equipped with a 420-nm cutoff filter. Hydrogen production was determined by an Aglient 6820 GC (TCD, 13× column, Ar carrier). The measurements of AQE were performed under the irradiation of monochromatic light with wavelength of 430, 490, 540, 590, 630, 730, and 800 nm. The AQE were finally obtained from the Eq. 7 [2] : 
    AQE = 2 × the number of evolved H_2 molecules/The number of incident photons× 100%
 (7) The STH efficiency was evaluated by using AM 1.5 G solar simulator as the light source and calculated as [2] 
    STH = Energy of generation of hydrogen by water splitting/Solar energy irradiating the reaction cell× 100%
 (8) Band-edge positions of the BP and Co-P/BP nanosheets To determine the absolute band-edge positions, we fabricated the BP and Co-P/BP nanosheets electrodes on fluorinated tin oxide (FTO) glass and measured their flat-band potentials, which were analyzed using the method reported before [55] . The variation of capacitance ( C ) with applied potential, therefore, can be expressed as [56] 
    1/C^2 = 2/ε·ε_0·e_0·A^2·N_D(E - E_FB - kT/e_0)
 (9) where C is the space charge capacitance. ε and ε 0 are the permittivity of the electrode and free space. e 0 , A , E , and E FB are elementary charge, electrochemical specific surface area, applied potential, flat-band potential, respectively. N D is the carrier density, k is the Boltzmann’s constant and T is the temperature. Generally, the potential measured against a Ag/AgCl reference can be converted as RHE potentials by [20] 
    E_FB(vs. RHE) = E_FB(Ag/AgCl) + E_AgCl + 0.059×pH
 (10) The pH value of the electrolyte is around 13, and E AgCl = 0.197 V. As a result, the flat-band positions of the BP and Co-P/BP nanosheets were calculated to be around −0.11 and −0.10 V vs. NHE (pH = 0), respectively. Furthermore, according to the XPS valence spectra (Supplementary Fig. 7 ), the VB energy levels of BP and Co-P/BP nanosheets are estimated to be ~0.51 and ~0.48 eV below the Fermi level. Therefore, the VB and CB are deduced to be −0.76 and 0.40 V for the BP, and −0.76 and 0.38 for the Co-P/BP vs. RHE, respectively. Preparation of working electrodes and electrochemical measurements Electrochemical experiments were carried out with a CHI660E electrochemical workstation in a conversional three-electrode systems composed of a Pt counter electrode, a reference electrode of saturated calomel electrode (SCE) and a working electrode. The working electrodes were fabricated by drop-coating water suspensions onto the precleared FTO glass or glassy carbon electrode (GCE) surface. Typically, catalyst powder (4 mg) was suspended in 15 ml ultrapure water, followed by ultrasonic treatment to form homogeneous solution for 30 min. Then, 0.55 ml of the above solution was dropped onto the precleaned GCE or FTO glass surface, followed by air-drying (loaded about 0.1 mg cm −2 ) before measurement. For comparisons, 0.5 mol L −1 of H 2 SO 4 aqueous solutions, pure water or H 2 O 2 aqueous solutions were used as the supporting electrolytes, respectively. The cathodic polarization curves were recorded on a linear sweep voltammetry technique with a scan rate of 50 mV s −1 . The cyclic voltammetry curves were tested with different sweep rate range from 10 to 150 mV s −1 , and scanning area from −0.5 to 0.5 V. The electrochemical impedance spectroscopy was measured at a frequency from 10 5 to 0.01 Hz. The Mott–Shottky curves were obtained by Impedance-potential technology at difference frequency. A 300-W Xe lamp equipped with an optical cutoff filter of 420 nm and output power of 100 mW cm −2 was used as light source. H 2 O 2 detection H 2 O 2 detection was carried out in 2.0 mL of the suspension, which was taken immediately after the irradiation. For each test, 0.5 mL of 1% o-tolidine in 0.1 M HCl (Alfa Aesar, 98%, without further purification) was dropped to the suspension [53] . In the presence of peroxides, a blue color is formed very quickly, indicating that the oxidation of o-tolidine. Subsequently, the dispersion was acidified with 1 M HCl (2 mL), which leads to the color of the solution to turn yellow. The yellow species is the protonated form of the two-electron oxidation product of o-tolidine (the reaction mechanism and solution color change are shown in Supplementary Fig. 24 ). The dispersion was quickly filtered through a 0.22 μm membrane filter and the absorption spectrum of the filtrate was immediately recorded on a UV–Vis spectrophotometer (Shimadzu, UV-2550). The absorption spectrum of the two-electron oxidized toluidine has a characteristic peak at 438 nm. EPR measurements EPR of radicals trapped by 5, 5-dimethyl-1-pyrroline N-oxide (DMPO) was measured with a Brucker EPR A200 spectrometer. The solution containing 0.1 mg mL −1 of the Co-P/BP nanosheets and 0.05 M of DMPO was vacuumed, followed by ventilating with argon for three times. Afterwards, the solution was added into a quartz cup inside the microwave cavity and irradiated by Xe lamp. The distance between the sample and the lamp was fixed to be 25 cm. The settings for the EPR measurements includes center field of 3486.70 G, sweep width of 100 G, microwave frequency of 9.82 GHz, modulation frequency of 200 kHz and power of 20.00 mW. Poisoning of the Co-P/BP nanosheets by H 2 O 2 To check the generated H 2 O 2 having a poison effect on the Co-P/BP nanosheets, a comparison experiment was carried out. In detail, 40 mg of the Co-P/BP nanosheets dispersed in suspension containing 150 mL of pure water and 2 mL of H 2 O 2 solution (50%, w/w). The change of the solution color was recorded and shown in Supplementary Fig. 26 . With increasing time, the color of the solution changed from brown to bright yellow and the solution pH was about 4–5 after 120 h, indicating that the generated H 2 O 2 has a poisoning effect on the Co-P/BP nanosheets. Therefore, how to remove generated H 2 O 2 is crucial during the photocatalytic reaction. Photo-electrochemistry study of H 2 O 2 decomposition To further prove the catalyst having no activity for H 2 O 2 decomposition, the electrochemical behavior of electrodes made by different catalysts was measured using cyclic voltammetry in 10 mM of H 2 O 2 solution under darkness. The electrochemical tests were carried out in a traditional three-electrode system consisting of the working electrodes of bare glassy carbon (GC) (black trace), BP (green trace) and Co-P/BP nanosheets (blue trace) modified GC electrodes, respectively. As shown in Supplementary Fig. 27a , the photocurrent exhibits decrease trend after injected high concentration H 2 O 2 , indicating the high concentration H 2 O 2 have a fatal for our system. Furthermore, Supplementary Fig. 27b and c clearly show that the modified BP and Co-P/BP nanosheets electrodes exhibit the basically similar onset potential and current at −0.90 V vs. SCE, indicating that both the Co-P/BP nanosheets and BP nanosheets basically have no catalytic activity toward H 2 O 2 decomposition. Furthermore, the photocurrent exhibits a decreasing trend with the increase of reaction time, compared with that without extra addition of H 2 O 2 . This indicates that a large amount of H 2 O 2 is bad for the stability of the catalyst. Thus, separation of H 2 O 2 generated during photocatalytic reaction is necessary for keeping the catalyst surviving. Data availability The data that support the findings of this study are available from the corresponding author on request.